Exfoliation of layered double hydroxides for enhanced oxygen evolution catalysis The oxygen evolution reaction is a key reaction in water splitting. The common approach in the development of oxygen evolution catalysts is to search for catalytic materials with new and optimized chemical compositions and structures. Here we report an orthogonal approach to improve the activity of catalysts without alternating their compositions or structures. Specifically, liquid phase exfoliation is applied to enhance the oxygen evolution activity of layered double hydroxides. The exfoliated single-layer nanosheets exhibit significantly higher oxygen evolution activity than the corresponding bulk layered double hydroxides in alkaline conditions. The nanosheets from nickel iron and nickel cobalt layered double hydroxides outperform a commercial iridium dioxide catalyst in both activity and stability. The exfoliation creates more active sites and improves the electronic conductivity. This work demonstrates the promising catalytic activity of single-layered double hydroxides for the oxygen evolution reaction. Water splitting is considered as an essential reaction to enable the storage of intermittent solar and wind energies in the form of chemical fuels, namely hydrogen and oxygen [1] . The oxygen evolution reaction (OER) is the bottleneck in water splitting. Even with state-of-the-art precious catalysts such as RuO 2 and IrO 2 , a substantial overpotential is required to drive the OER. The development of efficient, abundant and inexpensive OER catalysts is one of the main themes of current research in renewable energies [2] , [3] . Transition metal oxides and their derivatives are attractive catalyst candidates thanks to their diversity and potential stability. Nocera and co-workers [4] , [5] reported the high activity and stability of Co-phosphate and Ni-borate catalysts in neutral and weakly basic medium. Shao-Horn and co-workers [6] showed that perovskite Ba 0.5 Sr 0.5 Co 0.8 Fe 0.2 O 3−δ was an efficient OER catalyst in alkaline medium. In addition, mixed metal oxides of Fe, Co and Ni were reported to have good OER activity in alkaline medium [7] , [8] , [9] , [10] , often outperforming simple Co and Ni oxides and hydroxides. It has been proposed that in both crystalline metal oxides and amorphous Co-phosphate and Ni-borate catalysts, the active materials are layered hydroxides or oxyhydroxides composed of edge-sharing octahedral MO 6 layers [7] , [11] , [12] , [13] , [14] . Notwithstanding this progress, the current development of OER catalysts is focused on the discovery of new chemical compositions and structural phases; even with the help of useful descriptors and computational methods [6] , [15] , advances in this field are one-dimensional and often rely on fortuitous findings. Metal hydroxides and oxyhydroxides are composed of edge-sharing octahedral MO 6 layers ( Fig. 1a ). These layers are preserved in layered double hydroxides (LDHs). However, the presence of anions and water within the layers results in a larger inter-layer distance in LDHs ( Fig. 1b ). Although the OER activity of several LDHs has been studied [10] , [16] , [17] , [18] , that of single-layer nanosheets of LDHs ( Fig. 1c ) is not yet examined. Recently liquid exfoliation of layered materials has emerged as a transformative process in producing novel two-dimensional materials with drastically improved surface activity compared with their bulk, layered counterparts [19] , [20] , [21] , [22] , [23] , [24] , [25] , [26] . 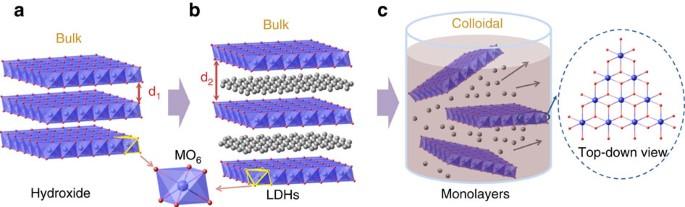Figure 1: Schematic representation of materials’ structures. (a) Layered hydroxides. d1is the inter-layer distance. (b) LDHs with inter-layer anions and water molecules. d2is the inter-layer distance, d2>d1. (c) Exfoliated LDH monolayers dispersed in a colloidal solution. Each single layer is composed of edge-sharing octahedral MO6moieties (M denotes a metal element). Metal atoms: purple spheres; Oxygen atoms: red spheres; Inter-layer anions and water molecules: grey spheres. Hydrogen atoms are omitted. Figure 1: Schematic representation of materials’ structures. ( a ) Layered hydroxides. d 1 is the inter-layer distance. ( b ) LDHs with inter-layer anions and water molecules. d 2 is the inter-layer distance, d 2 >d 1 . ( c ) Exfoliated LDH monolayers dispersed in a colloidal solution. Each single layer is composed of edge-sharing octahedral MO 6 moieties (M denotes a metal element). Metal atoms: purple spheres; Oxygen atoms: red spheres; Inter-layer anions and water molecules: grey spheres. Hydrogen atoms are omitted. Full size image In this work, we show that exfoliation of layered metal hydroxides leads to materials with the same chemical compositions but greatly enhanced OER activity. Single-layer nanosheets prepared from NiFe and NiCo LDHs exhibit higher catalytic activity than a state-of-the-art IrO 2 catalyst. The exfoliation also enables the first direct measurement of edge-sharing MO 6 octahedral layers, the putative active surface in metal oxides and hydroxides, detached from the bulk materials. While LDHs have been exfoliated for electrochemical applications such as electrodes for supercapacitors, batteries and sensors, the enhancement of activity in those applications is due to an increase in electrochemical surface area (ECSA) [21] , [22] , [23] . On the contrary, we show that the higher OER activity of exfoliated LDHs is mainly attributed to an increase in the number of active edge sites and to higher electronic conductivity. Fabrication of LDHs and their exfoliated nanosheets In this study, CoCo, NiCo and NiFe LDHs are used as representative LDH materials. The CoCo and NiCo LDHs with Br − anions were prepared via a topochemical approach, while the NiFe LDH with CO 3 2− anions was obtained by a hydrothermal process. Detailed description of experimental method is given in the Methods section. The X-ray Diffraction (XRD) patterns confirmed the LDH structure, exhibiting sharp peaks corresponding to the (00n) planes of LDHs ( Fig. 2a and Supplementary Fig. 1 ). The Transmission Electron Microscopy (TEM) ( Fig. 2b–d ) and Scanning Electron Microscopy images ( Supplementary Fig. 2 ) show the hexagonal shape of the bulk particles. The CoCo and NiCo LDHs are several micrometres in size, while the NiFe LDH is submicrometre in size. The Energy-dispersive X-ray Spectra confirmed the composition of the as-synthesized materials ( Fig. 2e ). According to the XRD patterns, the inter-layer distances in these LDHs are 70% larger than those of the corresponding hydroxides ( Supplementary Table 1 ). To further increase the inter-layer distance which is a prerequisite for successful exfoliation, inter-layer anion exchange was then conducted by dipping the as-prepared LDHs into concentrated aqueous solutions of target anions [27] , [28] . The appropriate anions are NO 3 − for CoCo and NiCo LDHs, and ClO 4 − for NiFe LDH. From CoCo and NiCo LDHs-Br − to the corresponding LDHs-NO 3 − , the inter-layer distance increased from 7.8 Å to 8.7 Å; from NiFe LDH-CO 3 2− to LDH-ClO 4 − , the inter-layer distance increased from 7.7 Å to 9.1 Å ( Supplementary Fig. 1 and Table 1 ). The successful anion exchange was confirmed by the Energy-dispersive X-ray Spectra results ( Supplementary Fig. 3 ). After anion exchange, the morphology and diameter of LDHs remained ( Supplementary Fig. 4 ). 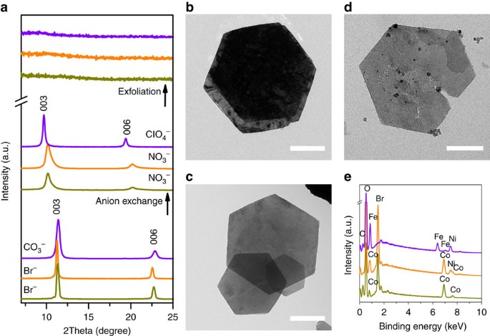Figure 2: Characterization of bulk LDHs. (a) XRD spectra. (b–d) TEM images of (b) CoCo LDH-Br−. Scale bar, 1 μm. (c) NiCo LDH-Br−. Scale bar, 1 μm. (d) NiFe LDH-CO32−. Scale bar, 150 nm. (e) Energy-dispersive X-ray Spectra. CoCo LDH: yellow-green lines; NiCo LDH: orange lines; NiFe LDH: purple lines. Figure 2: Characterization of bulk LDHs. ( a ) XRD spectra. ( b – d ) TEM images of ( b ) CoCo LDH-Br − . Scale bar, 1 μm. ( c ) NiCo LDH-Br − . Scale bar, 1 μm. ( d ) NiFe LDH-CO 3 2− . Scale bar, 150 nm. ( e ) Energy-dispersive X-ray Spectra. CoCo LDH: yellow-green lines; NiCo LDH: orange lines; NiFe LDH: purple lines. Full size image The increased inter-layer spacing after anion exchange allowed the delamination of the bulk LDHs to single-layer nanosheets. After being dispersed in purged formamide under stirring for 24 h, suspensions of bulk LDHs particles became clear solutions ( Fig. 3a ). The Tyndall effect observed upon irradiation of the solutions with a laser beam confirmed the colloidal nature of the solutions [28] , [29] , which was a first indication of the exfoliation of bulk LDHs into single layers. A further evidence of successful exfoliation was the absence of (00n) peaks in the XRD patterns ( Fig. 2a and Supplementary Fig. 5 ). The single-layer nanosheets were directly observed by TEM. A typical image of NiCo LDH single layer is shown in Fig. 3c while that of bulk NiCo LDH particle is shown in Fig. 3b for comparison. Analogous images of CoCo and NiFe LDHs and their exfoliated nanosheets are shown in Supplementary Fig. 6 . The exfoliated nanosheets had a faint contrast, consistent with their very thin nature. The Selected Area Electron Diffraction (insets in Fig. 3b,c ) are hexagonally arranged spots, indicating that the exfoliated nanosheets are still single crystalline, with the same phase as their original bulk LDHs. This result confirmed that single layers of the two-dimensional MO 6 network were delaminated from the bulk LDHs along the (00n) planes without a change of the basic structure of the layer. To further confirm the formation of single layers, exfoliated NiCo LDH nanosheets were dispersed on a silicon wafer for Atomic Force Microscopy (AFM, Fig. 3d ). The height profiles are shown in Fig. 3e . The thickness of the nanosheets was about 0.8 nm. This value is consistent with the thickness of a single layer of LDHs [29] , [30] . 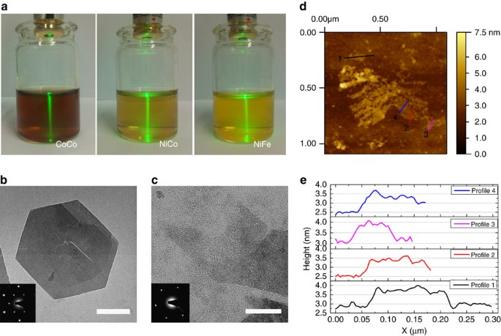Figure 3: Structural characterization of exfoliated LDH nanosheets. (a) Optical images of colloidal solutions of exfoliated nanosheets. Tyndall effect was visible when irradiated with a laser beam. (b) TEM images of bulk NiCo LDH nanoparticles. Inset is the corresponding Selected Area Electron Diffraction (SAED) pattern. Scale bar, 400 nm. (c) TEM images of exfoliated single-layer nanosheet of NiCo LDH. Scale bar, 100 nm. Inset is the corresponding SAED pattern where the spots can be indexed to crystalline plane family of {110}. (d) AFM image of exfoliated single-layer nanosheets of NiCo LDH. (e) Height profile of the exfoliated monolayer of NiCo LDH. The profiles 1, 2, 3 and 4 correspond to the numbered lines inFig. 3d, respectively. The average thickness is about 0.8 nm. Figure 3: Structural characterization of exfoliated LDH nanosheets. ( a ) Optical images of colloidal solutions of exfoliated nanosheets. Tyndall effect was visible when irradiated with a laser beam. ( b ) TEM images of bulk NiCo LDH nanoparticles. Inset is the corresponding Selected Area Electron Diffraction (SAED) pattern. Scale bar, 400 nm. ( c ) TEM images of exfoliated single-layer nanosheet of NiCo LDH. Scale bar, 100 nm. Inset is the corresponding SAED pattern where the spots can be indexed to crystalline plane family of {110}. ( d ) AFM image of exfoliated single-layer nanosheets of NiCo LDH. ( e ) Height profile of the exfoliated monolayer of NiCo LDH. The profiles 1, 2, 3 and 4 correspond to the numbered lines in Fig. 3d , respectively. The average thickness is about 0.8 nm. Full size image Oxygen evolution catalysis The exfoliated nanosheets of LDHs were then tested for electrochemical OER in 1 M KOH solutions. The catalysts were electrochemically pre-conditioned (30 cyclic voltammetric scans for CoCo and NiCo LDHs and galvanostatic oxidation for NiFe LDH) to reach a stable state ( Supplementary Figs 7, 8 and 9 ). Then the water oxidation activity was measured by linear sweep voltammetry. While bulk CoCo, NiCo and NiFe LDHs are decent OER catalysts in agreement with earlier reports [10] , [16] , [17] , Fig. 4a shows that the catalytic currents were shifted to significantly lower overpotentials upon exfoliation of bulk materials into nanosheets. Thus, the exfoliated nanosheets are better catalysts than their bulk counterparts. Three parameters were calculated to quantify the improvement of activity: the overpotential at a current density ( J ) of 10 mA cm −2 , the current density at an overpotential ( η ) of 300 mV and the Tafel slope. The current density of 10 mA cm −2 was chosen because it represents the current density from a device with 12% solar to hydrogen efficiency, which is at the upper end of a realistic device. 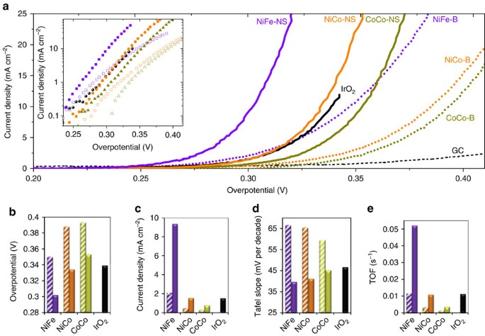Figure 4: Electrochemical behavior of LDH materials and IrO2nanoparticles. (a) Polarization curves. Inset shows the Tafel plots. Scan rate was 5 mV s−1. The loading was about 0.07 mg cm−2for LDH materials and 0.21 mg cm−2for IrO2nanoparticles. The electrolyte was 1 M KOH. (b) Overpotential required forJ=10 mA cm−2. Plots with error bar is shown inSupplementary Fig. 10. (c) Current densities atη=300 mV. (d) Tafel slopes. (e) TOF calculated from current atη=300 mV. CoCo LDH: yellow-green colour; NiCo LDH: orange colour; NiFe LDH: purple colour. Dash lines, hollow symbols and patterned columns: bulk LDHs (B); Solid lines, symbols and columns: exfoliated LDHs nanosheets (NS); Black lines, symbols and columns: IrO2nanoparticles; GC: glassy carbon electrode. Figure 4b shows that at J =10 mA cm −2 , the overpotentials were decreased by 40–54 mV upon exfoliation. Figure 4c shows that the current densities at η =300 mV were enhanced by 2.6-, 3.4- and 4.5-folds upon exfoliation of CoCo, NiCo and NiFe LDHs, respectively. The improved catalytic activity of exfoliated nanosheets was also reflected in their lower Tafel slopes ( Fig. 4d ). The Tafel slopes of exfoliated nanosheets of CoCo, NiCo and NiFe LDHs are 45, 41 and 40 mV per decade, respectively, while those of their bulk counterparts are 59, 65 and 67 mV per decade, respectively. The lower Tafel slopes of the nanosheet catalysts led to an even higher enhancement in OER activity by exfoliation at η >300 mV, because their current densities increased more rapidly with an increase of overpotentials. The fact that exfoliation decreases the Tafel slopes suggests that electron transport is more facile on single-layer nanosheets than in bulk LDHs. Figure 4: Electrochemical behavior of LDH materials and IrO 2 nanoparticles. ( a ) Polarization curves. Inset shows the Tafel plots. Scan rate was 5 mV s −1 . The loading was about 0.07 mg cm −2 for LDH materials and 0.21 mg cm −2 for IrO 2 nanoparticles. The electrolyte was 1 M KOH. ( b ) Overpotential required for J =10 mA cm −2 . Plots with error bar is shown in Supplementary Fig. 10 . ( c ) Current densities at η =300 mV. ( d ) Tafel slopes. ( e ) TOF calculated from current at η =300 mV. CoCo LDH: yellow-green colour; NiCo LDH: orange colour; NiFe LDH: purple colour. Dash lines, hollow symbols and patterned columns: bulk LDHs (B); Solid lines, symbols and columns: exfoliated LDHs nanosheets (NS); Black lines, symbols and columns: IrO 2 nanoparticles; GC: glassy carbon electrode. Full size image Among the three LDHs studied here, the catalytic activity has the order of NiFe>NiCo>CoCo for both exfoliated nanosheets and bulk LDHs. The activity of these non-precious materials was then compared with a state-of-the-art precious catalyst, IrO 2 ( Fig. 4 and Supplementary Fig. 11 ). Exfoliated nanosheets of NiFe and NiCo LDHs indeed outperformed IrO 2 nanoparticles, even at a comparatively lower loading (0.07 mg cm −2 for nanosheets and 0.21 mg cm −2 for IrO 2 ). These two nanosheet catalysts also exhibit comparable and often superior activity to the best known metal oxide catalysts ( Supplementary Table 2 ) [6] , [7] , [8] , [9] , [10] , [31] , [32] . The activity of exfoliated nanosheets was also expressed in apparent turnover frequencies (TOFs), assuming that all the metal ions in the nanosheets were active. Figure 4e shows that nanosheets of NiFe and NiCo LDHs have TOFs of 0.05 and 0.01 s −1 at η =300 mV, respectively. These are the minimum values for TOFs. The TOFs can be estimated by another two methods. Taking exfoliated NiFe LDH as an example, and based on the Ni content detected by Inductively Coupled Plasma Optical Emission Spectrometry, the TOF was calculated to be about 0.11 s −1 . Based on the Ni content calculated from the total charge of the Ni 2+ /Ni 3+ redox wave in the cyclic voltammogram (CV; Supplementary Fig. 9 ), the TOF was calculated to be about 0.24 s −1 . The latter is comparable to the value obtained by Trotochaud et al . 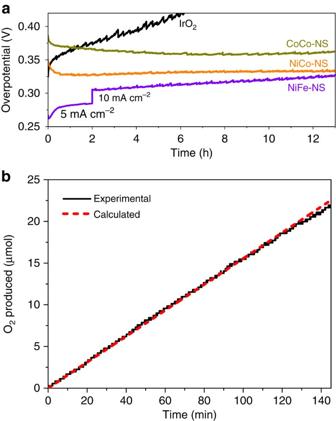Figure 5: Long-term stability and Faradaic efficiency. (a) Chronopotentiometric measurements atJ=10 mA cm−2; for exfoliated NiFe LDH, current density was kept atJ=5 mA cm−2for the first 2 h until the potential was stable. NS denotes nanosheets. (b) Calculated versus actual oxygen production catalyzed by exfoliated NiCo LDH at a constant current of 1 mA after a pretreatment of 35 min. The calculated value represent the expected amount of O2assuming a quantitative Faradaic yield for O2formation. [7] The stability of nanosheet catalysts was tested at a constant current density J of 10 mA cm −2 for 13 h. Figure 5a shows that nanosheets of CoCo and NiCo LDHs have good electrochemical stability, as the overpotential remained nearly constant during 13 h. Nanosheets of NiFe LDH gradually fell off the electrode if electrolyzed at J =10 mA cm −2 for an extended time. If the electrolysis current density was set to 5 mA cm −2 for the first 2 h, and was then switched to 10 mA cm −2 , a relative stable behaviour was observed for 10 h. The stability test was also conducted on IrO 2 . As shown in Fig. 5a , the overpotential for maintaining a J of 10 mA cm −2 increased from 325 to 419 mV during 6 h, indicating lower stability of IrO 2 compared with the nanosheets. Figure 5: Long-term stability and Faradaic efficiency. ( a ) Chronopotentiometric measurements at J =10 mA cm −2 ; for exfoliated NiFe LDH, current density was kept at J =5 mA cm −2 for the first 2 h until the potential was stable. NS denotes nanosheets. ( b ) Calculated versus actual oxygen production catalyzed by exfoliated NiCo LDH at a constant current of 1 mA after a pretreatment of 35 min. The calculated value represent the expected amount of O 2 assuming a quantitative Faradaic yield for O 2 formation. Full size image The NiFe LDH nanosheets were also deposited on a porous Ni foam (loading: 1 mg cm −2 ) and the chronoamperometric measurement at η =300 mV was conducted ( Supplementary Fig. 12 ). The current density was constant at about 24 mA cm −2 . This result suggests the nanosheets of NiFe LDH are intrinsically stable under OER conditions. The NiCo LDH nanosheets were also deposited on a porous Ni foam (loading: 1 mg cm −2 ) ( Supplementary Fig. 13 ). The resulting electrode gave a stable current density of 23 mA cm −2 at η =300 mV. To confirm that the oxidation currents were associated with water oxidation, the amount of oxygen produced during OER electrolysis at 14 mA cm −2 was measured for the NiCo nanosheet catalyst. The catalyst has a nearly quantitative Faradaic efficiency after an induction period of 35 min ( Fig. 5b and Supplementary Fig. 14 ). The induction period might be attributed to the pre-condition of catalyst and the dissolution of the initially produced O 2 in the electrolyte solution. Surface area is an important factor in catalysis; the increase of surface area is often primarily responsible for enhanced catalytic activity after nanostructuring. The origin of the enhanced OER activity by exfoliation described here was therefore probed by comparing the catalytic activity and ECSA of metal hydroxides, bulk LDH and their exfoliated nanosheets. Transformation from NiCo hydroxide to bulk NiCo LDH-NO 3 − resulted in a 2.5 times increase in current density at η =350 mV, and the exfoliation resulted in a further 6.5 times increase ( Fig. 6a ). The ECSA of these materials were estimated from the electrochemical double-layer capacitance (C dl ) of the catalysts ( Fig. 6b ). The linear slope of capacitive current versus scan rate, equivalent to twice of the double-layer capacity C dl , was used to represent the ECSA [33] , [34] . From NiCo hydroxides to NiCo LDH-NO 3 − , the ECSA increased by 13-fold. This increase is attributed to the enhanced anion exchangeability between the layers in LDH as the inner layer surface is now electrochemically accessible. Exfoliation of LDH resulted in only a 30% further increase in ECSA. The increase is small because the inner layer surface in bulk LDH is already largely accessible in electrochemical capacity measurements. The 13-fold increase in ECSA from NiCo hydroxides to NiCo LDH is the main contributor to the 2.5-fold increase in catalytic activity. However, the 30% further increase in ECSA upon exfoliation of bulk NiCo LDH-NO 3 − cannot account for the 6.5-fold increase in activity after exfoliation. 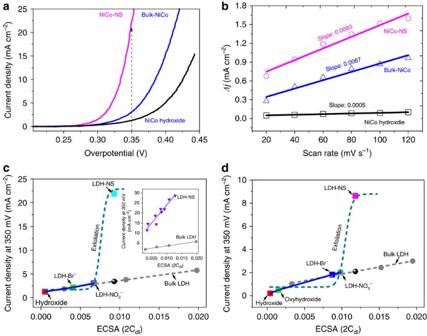Figure 6: Change of catalytic activity and ECSA. (a) Polarization curves of NiCo hydroxide, NiCo LDH-NO3−, and nanosheets (NS) of NiCo LDH. Scan rate was 5 mV s−1. Loading was about 0.07 mg cm−2. The arrow points to the current density atη=350 mV. (b) Charging current density differences (Δj=ja−jc) plotted against scan rates. The linear slope, equivalent to twice of the double-layer capacitance Cdl, was used to represent the ECSA. (c) Current density atη=350 mV plotted against ECSA (2Cdl) for NiCo-based materials. (d) Current density atη=350 mV plotted against ECSA for CoCo-based materials. Solid square (coloured incandd): hydroxides, oxyhydroxides, bulk LDHs with different inter-layer anions and LDH nanosheets at the same loading (0.07 mg cm−2); Grey solid sphere (incandd): bulk LDH-NO3−at different loadings; Black solid sphere (incandd): estimated activity of bulk LDH-NO3−with the same ECSA as LDH nanosheets based on the fitting line; Solid triangle (inset inc): nanosheets of NiCo LDH at different loadings. Figure 6: Change of catalytic activity and ECSA. ( a ) Polarization curves of NiCo hydroxide, NiCo LDH-NO 3 − , and nanosheets (NS) of NiCo LDH. Scan rate was 5 mV s −1 . Loading was about 0.07 mg cm −2 . The arrow points to the current density at η =350 mV. ( b ) Charging current density differences (Δ j = j a − j c ) plotted against scan rates. The linear slope, equivalent to twice of the double-layer capacitance C dl , was used to represent the ECSA. ( c ) Current density at η =350 mV plotted against ECSA (2C dl ) for NiCo-based materials. ( d ) Current density at η =350 mV plotted against ECSA for CoCo-based materials. Solid square (coloured in c and d ): hydroxides, oxyhydroxides, bulk LDHs with different inter-layer anions and LDH nanosheets at the same loading (0.07 mg cm −2 ); Grey solid sphere (in c and d ): bulk LDH-NO 3 − at different loadings; Black solid sphere (in c and d ): estimated activity of bulk LDH-NO 3 − with the same ECSA as LDH nanosheets based on the fitting line; Solid triangle (inset in c ): nanosheets of NiCo LDH at different loadings. Full size image While NiCo LDH-Br − and CoCo LDH-Br − were not suitable for exfoliation due to a small inter-layer distance, their catalytic activity and ECSA were also measured as additional reference points. Figure 6c shows that there is a linear correlation between the activity and ECSA for NiCo hydroxide, NiCo LDH-Br − and NiCo LDH-NO 3 − (at the same loading; blue line); similar linear correlation exists for CoCo hydroxide, CoCo oxyhydroxide, CoCo LDH-Br − and CoCo LDH-NO 3 − (blue line, Fig. 6d ). This correlation indicates that for hydroxide and bulk LDHs, the difference in catalytic activity is mainly due to the difference in accessible surface areas. To further confirm this, the loading of NiCo LDH-NO 3 − and CoCo LDH-NO 3 − were varied and their catalytic activity and ECSA were measured. Figure 6c,d show that the activity and ECSA again are linearly correlated for the same LDH at different loadings (grey lines). Importantly, the slopes of blue and grey lines are similar. These lines can then be used to predict the ‘intrinsic’ activity of this type of materials assuming surface area as the sole variable. Similar correlation was found for NiFe LDHs ( Supplementary Fig. 15 ). Upon exfoliation, the catalytic activity increased dramatically while the ECSA only changed slightly ( Fig. 6c,d and Supplementary Fig. 15 ). The expected activity according to the linear correlation described above (represented by black solid spheres in the figures) was much lower than that observed for the exfoliated nanosheets of LDHs. This result clearly excludes increased ECSA as the main contributor to the significant enhancement of OER activity by exfoliation. To further verify this, we measured the activity and ECSA of exfoliated nanosheets at different loadings. A linear correlation between the activity and ECSA is again found within these nanosheets (inset in Fig. 6c ). However, the slope is much larger than that of bulk hydroxide and LDHs. This result indicates that the exfoliated nanosheets have higher intrinsic catalytic activity. The higher intrinsic activity of exfoliated nanosheets might be due to a larger number of active sites. To verify this, the morphologies of nanosheets and the bulk LDHs were further examined. According to TEM ( Fig. 3b–d and Supplementary Fig. 6 ), the exfoliated nanosheets are smaller in dimension. For CoCo and NiCo LDHs, exfoliation reduced the size from 1–5 μm to less than 500 nm. For NiFe LDH, while some nanosheets retained the size of the bulk LDH (200–500 nm), others were smaller. Fortuitously, some samples of incomplete exfoliation were obtained. Supplementary Figure 16 shows the TEM image of a NiCo sample, which might be considered as a snap shot of the transition between the bulk LDH to exfoliated nanosheets. According to this image, exfoliation not only results in single layers, but also reduces the size of the layer. The reduction in size should increase significantly the edge lengths while maintaining a similar surface area. The edges are expected to contain open coordination sites that might be the active sites for water oxidation. While this hypothesis is consistent with the observations, the rigorous identification and confirmation of the active sites of the exfoliated nanosheets will require a dedicated study to correlate the edge length with activity in the near future, as done for MoS 2 nanocrystals for hydrogen evolution [35] . In addition to higher catalytic current densities, the improvement of OER activity by exfoliation is also reflected in the lower Tafel slopes ( Fig. 4d ). The decrease in Tafel slope might be due to an increase in electron conductivity [36] . Bulk LDHs suffer from low conductivity due to the large inter-layer distance. Previously, it was shown that incorporation of graphene oxide into the LDH layers enhanced the conductivity of LDH for supercapacitor applications [21] . In the current case, exfoliation transforms the rigid multilayers of LDH into single-layer nanosheets. When assembled on a conducting substrate, these stacked nanosheets are expected to have better electron transport property than the bulk LDHs. Thus, improved conductivity might be a second contributor for the enhanced activity. The results presented here can be compared to a recent study utilizing alternative approach to obtain thin LDH layers for OER. Dai and co-workers [10] were able to grow thin NiFe LDH particles that were several-layer thick (4 nm). These particles exhibited OER activity superior to bulk NiFe LDH ( Supplementary Table 2 ), but inferior to the exfoliated nanosheets of NiFe LDH (our data). The several-layer thick NiFe LDH can be considered as partially exfoliated LDH; it has a similar size as the fully exfoliated LDH, but should have lower electronic conductivity. It was also shown that when grown on carbon nanotubes (CNT), the activity of several-layer thick NiFe LDH was further enhanced. While it is difficult to compare the activity of single and hybrid materials, the enhancement in activity was attributed partially to higher conductivity of the CNT-LDH hybrid, and partially to a special interaction between CNT and LDH that might alter the electronic structure of LDH. Despite the different approach, the results of the study by Dai and co-workers [10] are consistent with our proposal that more abundant edge sites and higher conductivity are responsible for higher activity of exfoliated LDH nanosheets. In this regard, this work can be distinguished from earlier studies of exfoliation of LDHs for applications such as capacitors, batteries and sensors [21] , [22] , [23] . In those studies, exfoliation mostly increases the ECSAs. Likewise, the increased contact area is largely responsible for enhanced performance of exfoliated metal chalcogenide nanosheets as sensors [19] , [20] , [25] . On the other hand, the enhancement in OER activity presented here is mainly attributed to the improvement of chemical and electronic properties of exfoliated LDH nanosheets. Jin and co-workers [34] reported an exfoliation approach to develop hydrogen evolution catalyst. They exfoliated MoS 2 to transform the less active 2H-phase to the more active 1T-phase. The enhanced activity of the 1T-phase was attributed to higher conductivity and active site density. The present exfoliation of LDHs, however, does not involve phase transition. Xie and co-workers [26] prepared single-layered ZnSe nanosheets which exhibited unique electronic property relative to bulk ZnSe, which is non-layered. The ZnSe nanosheets had much higher activity in photocatalytic-water oxidation under ultraviolet light than the bulk sample. To further elucidate the mechanism for the enhanced catalytic activity of the exfoliated LDH nanosheets, we plan to compare the structures and electronic properties of exfoliated and bulk LDHs by advanced spectroscopic and computational methods. The possible structural changes in surface distortion and interatomic distances upon exfoliation might be detected by synchrotron-radiation X-ray adsorption fine structure spectroscopy, which has been previously applied to probe the structural changes due to exfoliation of layered metal chacogenides [24] , [26] , [37] , [38] . The structural change upon exfoliation will also be computed using density functional theory-based methods. The electronic properties, especially the energies of valance orbitals, will be measured by ultraviolet photoelectron spectroscopy. The band structures will be calculated using density functional theory. These combined experimental and computational measurements will hopefully yield insights into the physical origins of the enhanced catalytic activity upon exfoliation of bulk LDHs. In summary, we show that exfoliated single-layer nanosheets of LDHs are highly active electrocatalysts for OER, competing favourably against the costly IrO 2 catalyst. The significantly higher catalytic activity of the nanosheets compared with the bulk LDHs originated mainly from the increase in active site density and conductivity while maintaining similar ECSAs. Our study demonstrates a new ‘top-down’ approach in the development of OER catalysts. This approach should be applicable to many of the newly discovered metal oxide OER catalysts, adding a new dimension in this urgent area of energy research. Fabrication of CoCo and NiCo LDHs A topochemical approach was used to fabricate CoCo and NiCo LDHs by oxidizing corresponding hydroxides in Br 2 solution [28] . In 500 ml of deionized water, 2.5 mmol of cobalt chloride (CoCl 2 ·6H 2 O, ACS reagent, 98–102%, Acros) and 45 mmol of hexamethylenetetramine (HMT, 99%, Sigma-Aldrich) were dissolved. The solution was refluxed at 95 °C for 5 h under continuous magnetic stirring and a N 2 atmosphere. Pink powder of brucite Co(OH) 2 was collected by centrifuging the reaction mixture at a speed of 3,000 r.p.m for 10 min. The powder was washed with deionized water and ethanol, and dried at room temperature. For Ni 1/3 Co 2/3 (OH) 2 hydroxides, 1.25 mmol of nickel chloride (NiCl 2 , anhydrous for analysis, Merck Schuchardt OHG ) was firstly dissolved in 500 ml deionized water, and then 2.5 mmol of cobalt chloride (CoCl 2 ·6H 2 O) and 45 mmol of HMT were added. The subsequent procedure was the same as that for the synthesis of Co(OH) 2 hydroxides. Light-pink powder of brucite-like Ni 1/3 Co 2/3 (OH) 2 was obtained. The as-obtained hydroxides were topochemically oxidized to LDHs-Br. Hundred milligrams of Co(OH) 2 was dispersed in a solution of 0.269 ml of Br 2 (99+%, extra pure, Acros) and 83 ml of acetonitrile (Merch KGaA), while 100 mg Ni 1/3 Co 2/3 (OH) 2 was dispersed in a solution of 0.185 ml of Br 2 and 54 ml of acetonitrile. These mixtures were sealed in an airtight-capped flask and magnetically stirred for 1 day for Co(OH) 2 and 5 days for Ni 1/3 Co 2/3 (OH) 2 . The powders were recovered by centrifugation at a speed of 3,000 r.p.m for 10 min, washed with anhydrous ethanol for three times and dried at room temperature. The as-obtained blackish-brown and yellow-green powders were CoCo LDH-Br − (chemical formula: Co II 2/3 Co III 1/3 (OH) 2 Br 1/3 ·0.4H 2 O) and NiCo LDH-Br − (chemical formula: Ni II 1/3 Co II 1/3 Co III 1/3 (OH) 2 Br 1/3 ·0.5H 2 O). Anion exchange from Br − to NO 3 − was conducted via an ethanol-assisted anion-exchange method. Hundred milligrams of LDHs-Br − was dispersed into an 80 ml purged ethanol/water (1:1 v/v) solution of 1.5 M sodium nitrate (extra pure, Acros). The mixture was then mechanically stirred for 24 h under a N 2 atmosphere. The products were centrifuged at a speed of 3,000 r.p.m for 10 min, washed with purged deionized water and ethanol, and air-dried at room temperature. To exfolicate the LDHs, 50 mg of the powder (CoCo or NiCo LDHs-NO 3 − ) was dispersed in 100 ml of degassed formamide (ACS reagent, 99.6%, Acros) by sonication for 10 min, and then mechanically stirred under a N 2 atmosphere for 24 h. A Clear colloidal solution was formed. The Tyndall effect when irradiated with a laser beam confirmed the exfoliation to single LDHs layers. Fabrication of NiFe LDH A hydrothermal process was applied by using urea and triethanolamine (TEA, Sigma-Aldrich) as ammonium releasing reagent and chelating agent, respectively [29] . In a typical procedure, nickel nitrate (Ni(NO 3 ) 2 ·6H 2 O, ≥97%, Sigma-Aldrich) and iron nitrate (Fe(NO 3 ) 3 ·9H 2 O, ≥98%, Sigma-Aldrich) were dissolved in 200 ml of deionized water with TEA, to form a solution with a total metal cation concentration of 20 mM. The ratio of Ni 2+ and Fe 3+ were about 3:1, and the concentration of TEA was 2.5 times of that of Fe 3+ in the final solution. Then 7.0 mmol of urea and 200 ml of deionized water were added to the solution and magnetically stirred for 1 h. The above solution (80 ml) was transferred to a stainless-steel Teflon-lined autoclave. After being kept in a preheated oven at 150 °C for 2 days, the autoclave was cooled down naturally to room temperature. The resulting yellowish powder was collected by centrifugation at a speed of 3,000 r.p.m for 10 min. After washing with ethanol for three times and drying at room temperature, yellowish powder (chemical formula: Ni II 3/4 Fe III 1/4 (OH) 2 (CO 3 ) 1/8 ·0.8H 2 O) was obtained. Anion exchange was carried out in a solution containing an excess of the target anions [27] . Sodium chloride (NaCl, 1 M) and HCl (4 mM) solution were used for Cl − anion exchange. In a typical procedure, about 100 mg of the powder was dipped into a 100 ml of purged solution, sonicated for 5 min and mechanically stirred under a N 2 atmosphere for 1 day. The yellowish powder was centrifuged at a speed of 3,000 r.p.m for 10 min, and washed with purged deionized water and ethanol and finally dried at room temperature. To obtain NiFe LDH-ClO 4 − , the as-obtained NiFe LDH-Cl − powder was further exchanged in a solution of 2.5 M sodium perchlorate (NaClO 4 ·H 2 O, ACS reagent, ≥98.0% (T), Sigma-Aldrich) and 2.5 mM HCl. For the exfoliation, 50 mg of the powder (NiFe LDH-ClO 4 − ) was dispersed in 100 ml of degassed formamide by sonication for 10 min and then mechanically stirred under a N 2 atmosphere for 24 h. A yellowish translucent colloidal suspension was formed. The Tyndall effect when irradiated with a laser beam confirmed the exfoliation to single LDHs layers. Structural characterization XRD measurements were carried out on an X'Pert Philips diffractometer in Bragg-Brentano geometry with CuKα1 radiation and a fast Si-PIN multi-strip detector (0.1540, nm). For the XRD measurements, the samples were well dispersed on fluorine-doped tin oxide. Inductively Coupled Plasma Optical Emission Spectrometry analysis was performed on an Optima 2000 spectrometer (Perkin-Elmer). Standard solutions (TraceCERT) were purchased from Fluka (Sigma-Aldrich) and were used for calibration. Scanning Electron Microscopy secondary electron images were taken in a Phillips (FEI) XLF-30 FEG scanning electron microscope. TEM images were taken on a Philips (FEI) CM12 transmission electron microscope with a LaB 6 source operated at 100-kV accelerating voltage. AFM was performed on a Veeco NanoScope IIIA AFM instrument (Digital instruments, Santa Barbara, CA, USA) in tapping mode. AFM samples were prepared by dispersing NiCo LDH colloids on silicon substrates for 30 min, washing with deionized water and drying at 125 °C for 10 min. Electrode preparation For bulk LDHs and IrO 2 nanoparticles, 5 mg of powders were dispersed in 10 ml of deionized water and sonicated in an ultrasonic water bath. For exfoliated nanosheets of LDHs, the colloids were used directly. Glassy carbon disk electrodes with a diameter of 3 mm were used. They were polished with two different alpha alumina powder (1.0 and 0.3 μm from CH instruments) suspended in deionized water on a Nylon polishing pad (CH instruments), and with gamma alumina powder (0.05 μm from CH instruments) suspended in distilled water on a micro-cloth polishing pad (CH instruments). After the first and second stages of cleaning, the electrodes were thoroughly rinsed with deionized water. Before being loaded with catalysts, the electrodes were also cleaned in acetone by sonication for about 10 s. Ten microlitres of catalysts (colloids or suspensions) were then drop-casted on a glassy carbon disk electrode and the solvent was allowed to be evaporated at 125 °C. Ni foam (thickness: 1.6 mm) was purchased from Good Fellow Cambridge Limited. Before testing, the Ni foam was pretreated by 30 cycles of cyclic voltammetry between 0.3 and 0.75 V versus Hg/HgO in 1 M KOH. Pretreated Ni foam was drop-casted with colloidal catalysts at the loading of 1 mg cm −2 (loading area: 0.0625, cm 2 ). Electrochemical tests Electrolysis experiments were performed in a H-shaped cell. The platinum counter electrode was separated from the solution through a porous glass frit and this whole assembly was inserted into one side of the H cell. The modified working electrode was inserted in the other side of the cell, together with a magnetic stirring bar and a Luggin capillary. Electrochemical characterization was carried out in 1 M KOH electrolytes (1 mol l −1 (1 N), Merck KGaA). A Hg/HgO reference electrode with 1 M KOH filling solution was used throughout the experiments. Before test, the reference electrode was measured against another unused Hg/HgO reference electrode stored in 1 M KOH. All the potentials were measured against this Hg/HgO (1 M KOH) that has a potential of 0.098 V versus the normal hydrogen electrode, except for the O 2 evolution experiments. The equilibrium potential for oxygen evolution at any given PH is therefore (1.23−0.098−0.059 × PH) V versus Hg/HgO. Ohmic drop correction was performed using the current interrupt method by the potentiostat. Measurements were carried out using a Gamry Reference 3,000. Calibration of the potential was done by measuring the reversible hydrogen electrode potential using a Pt electrode under a H 2 atmosphere in the same electrolyte. CVs were recorded between 0.3 and 0.65–0.75 V versus Hg/HgO in 1 M KOH. Chronopotentiometric measurements were recorded at the current density of 10 mA cm −2 . For CoCo and NiCo LDHs and IrO 2 nanoparticles, CVs were recorded for 30 cycles when the oxygen evolution currents showed negligible change (scan rate: 10 mV s −1 ). Following these, five cycles of linear scan voltammograms (LSV) were measured (scan rate: 5 mV s −1 ), and then the ECSA were determined according to the method described below. For NiFe LDH, chronopotentiometric measurements at J =10 mA cm −2 were recorded until the potential was stable. Following this, five cycles of LSV were then measured (scan rate: 5 mV s −1 ), and the ECSA was determined. Tafel slopes were calculated from the LSV curves at the current density range of 1–10 mA cm −2 . ECSA was determined by measuring the capacitive current associated with double-layer charging from the scan-rate dependence of CVs. The ECSA was measured on the same working electrodes. For this, the potential window of CVs was 0.3–0.4 V versus Hg/HgO (1 M KOH). The scan rates were 20, 40, 60, 80 and 100 mV s −1 . The double-layer capacitance (C dl ) was estimated by plotting the Δj ( j a − j c ) at 0.35 V versus Hg/HgO (1 M KOH) against the scan rate. The slope is twice of the double-layer capacitance C dl . For samples loaded on porous Ni foam, chronoamperometric measurements were done at η =300 mV. The TOF value is calculated from the equation: Where J is the current density at a given overpotential (for example, η =300 mV), A is the surface area of the electrode, F is the Faraday constant, and m is the number of moles of metal on the electrode. Since there was no Ni II /Ni III redox peak for CoCo and NiCo LDHs, the Co atoms are assumed to be accessible for catalyzing the OER. For NiFe mixed metal oxides, Ni atoms were normally regarded as the active sites and herein there were obvious Ni II /Ni III redox peaks in the CVs. So for NiFe LDH, all the Ni atoms are assumed to be accessible for catalyzing the OER. The measurements of O 2 were performed using an Ocean Optics Multifrequency Phase Fluorimeter (MFPF-100) with a FOXY-OR 125 probe. A linear two-point calibration curve was created using air (20.9% O 2 ) and a sealed glass cell that had been purged with N 2 for more than 2 h (0% O 2 ). Electrolysis experiments were performed in an airtight H-shaped cell. The platinum counter electrode was inserted into one side of the cell. The modified working electrode, an Ag/AgCl reference electrode (has a potential of 0.197 V versus normal hydrogen electrode) and a magnetic stirring bar were inserted in the other side. The cell was filled with 1 M KOH solution until the headspace of the compartment containing the working electrode was about 6.3 ml. The oxygen probe was inserted into this headspace. The cell was purged with nitrogen for 20 min, and the O 2 concentration in the headspace was then monitored for 60 min to establish a baseline. A constant oxidation current of 1 mA was passed for 180 min. The faradaic yield was calculated from the total amount of charge Q (C) passed through the cell and the total amount of oxygen produced n O2 (mol). Q = t /1,000 (C), where t is the time (s) for the constant oxidation current. The total amount of oxygen produced was measured using the MFPF-100 with a FOXY 125 probe. Assuming that four electrons are needed to produce one O 2 molecule, the Faradaic efficiency can be calculated as follows: Faradaic efficiency=4F × n O 2 / Q= 4,000 F × n O 2 / t , where F is the Faraday constant. How to cite this article: Song, F. and Hu, X. Exfoliation of layered double hydroxides for enhanced oxygen evolution catalysis. Nat. Commun. 5:4477 doi: 10.1038/ncomms5477 (2014).